Self-assembled nanoscale coordination polymers with trigger release properties for effective anticancer therapy Nanoscale coordination polymers (NCPs) are self-assembled from metal ions and organic bridging ligands, and can overcome many drawbacks of existing drug delivery systems by virtue of tunable compositions, sizes and shapes, high drug loadings, ease of surface modification and intrinsic biodegradability. Here we report the self-assembly of zinc bisphosphonate NCPs that carry 48±3 wt% cisplatin prodrug and 45±5 wt% oxaliplatin prodrug. In vivo pharmacokinetic studies in mice show minimal uptake of pegylated NCPs by the mononuclear phagocyte system and excellent blood circulation half-lives of 16.4±2.9 and 12.0±3.9 h for the NCPs carrying cisplatin and oxaliplatin, respectively. In all tumour xenograft models evaluated, including CT26 colon cancer, H460 lung cancer and AsPC-1 pancreatic cancer, pegylated NCPs show superior potency and efficacy compared with free drugs. As the first example of using NCPs as nanotherapeutics with enhanced antitumour activities, this study establishes NCPs as a promising drug delivery platform for cancer therapy. Our understanding of cancer biology has progressed enormously in the past 20 years [1] , and yet mortality rates for many cancers have changed very little. The therapeutic efficacy of many clinically used anticancer drugs, particularly conventional chemotherapeutics, is limited by their inability to preferentially accumulate in tumour tissues [2] , [3] . Most chemotherapeutics are therefore administered at high doses to compensate for non-ideal biodistributions, which can lead to severe side effects [4] , [5] . Such dose-limiting side effects prevent the complete eradication of cancer in a patient, thus allowing the recurrence of cancer and the development of drug resistance [6] , [7] . For example, cisplatin is the most commonly used chemotherapeutic for treating testicular, lung, breast, bladder, ovarian, and head and neck cancers [4] , [8] , [9] . However, cisplatin causes numerous side effects, such as nephrotoxicity, which severely limit its clinical utility. Oxaliplatin was developed to treat gastric cancers, but its efficacy is also compromised by its dose limit toxicity, including peripheral neuropathy and neurotoxicity [10] . Therefore, the broader scientific and pharmaceutical community is in need of novel strategies for selective delivery of chemotherapeutics to tumour tissues. The development of such strategies will lead to enhanced therapeutic efficacy that will directly benefit cancer patients. Nanoparticles have recently emerged as a promising platform for the selective delivery of chemotherapeutics to cancer [3] , [11] . Such nanotherapeutics can have prolonged blood circulation times to allow for preferential tumour accumulation by taking advantage of their enhanced permeation and retention in the leaky vasculatures of tumour tissues [12] . Over the past two decades, many nanoparticle platforms, including liposomes [13] , [14] , [15] , polymeric micelles [16] , [17] , [18] , organic polymers [19] , [20] , [21] , [22] , [23] , [24] , dendrimers [25] , metal and metal oxide [26] , [27] , [28] , and mesoporous silica [29] , [30] , [31] have been developed for the delivery of chemotherapeutics to cancer. These intensive studies have led to successful clinical translation of several nanotherapeutics since 1995, including doxorubicin (Doxil), daunorubicin (Daunoxome), amphotericin B (Ambisome) and cytarabine (Depocyte). However, optimal nanotherapeutics have yet to be developed because each of the existing delivery systems has its own limitations; for example, most of the clinically used nanotherapeutics are liposomal formulations, which are intrinsically less amenable to encapsulate hydrophilic drugs. Nanoscale coordination polymers (NCPs) are constructed from metal-connecting points and organic bridging ligands via self-assembly processes [32] , [33] . We believe that NCPs can combine the advantages of both organic nanoparticles, such as compositional tunability, biodegradability and high drug loadings, and those of inorganic nanoparticles, such as well-defined particle morphologies and ease of surface functionalization, to afford an entirely new drug delivery platform. Although NCPs were previously examined as potential vehicles for delivering imaging agents and chemotherapeutics [34] , [35] , [36] , they have not yet been shown to be effective anticancer therapeutics in vivo . Here we report the development of a novel, self-assembled zinc bisphosphonate NCP platform for the selective delivery of cisplatin and oxaliplatin to tumours. Two bisphosphonate ligands based on cisplatin and oxaliplatin prodrugs are used to construct robust NCPs with trigger release kinetics. The NCPs are pegylated to further stabilize the particles and to allow for long blood circulation times. Both NCP particles demonstrate enhanced antitumour activity when compared with free drugs in three different tumour xenograft models. Self-assembly and characterization of Zn bisphosphonate NCPs Previously reported NCP-based nanotherapeutics use non-biocompatible metal ions and do not exhibit adequate stability for in vivo applications [37] , [38] . There are recent reports on in vivo evaluations of NCPs, but the unfavourable pharmacokinetics (pKs) and non-biocompatibility of these systems have greatly limited their applications in vivo [39] , [40] . We explored Zn(II)-bisphosphonate NCPs in this work to enhance particle stability [41] and reduce excipient toxicity. Bisphosphonic acids containing cisplatin and oxaliplatin prodrugs, L 1 -H 4 and L 2 -H 4 ( Fig. 1a ), were synthesized by treating Pt(NH 3 ) 2 Cl 2 (OH) 2 and Pt(dach)Cl 2 (OH) 2 (dach= R , R -diaminocyclohexane) with diethoxyphosphinyl isocyanate followed by deprotection of the phosphonate esters with bromotrimethylsilane ( Supplementary Figs 1–3 and Supplementary Methods ). 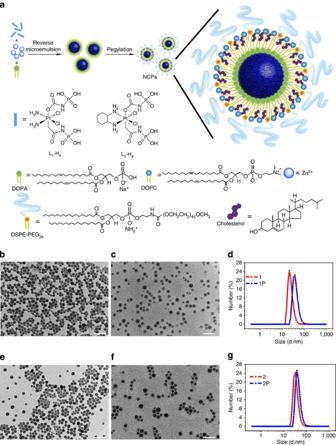Figure 1: Schematic illustration and TEM images of NCPs. (a) General procedure for self-assembly of NCPs with lipid and PEG coatings. TEM images of (b)1; (c)1P; (e)2; (f)2P. Size distribution of1(d) and2(g) measured by DLS. Scale bars, 100 nm. Figure 1: Schematic illustration and TEM images of NCPs. ( a ) General procedure for self-assembly of NCPs with lipid and PEG coatings. TEM images of ( b ) 1 ; ( c ) 1P ; ( e ) 2 ; ( f ) 2P . Size distribution of 1 ( d ) and 2 ( g ) measured by DLS. Scale bars, 100 nm. Full size image Zn(II) bisphosphonate NCP containing the cisplatin prodrug, 1 , was prepared by vigorously stirring a mixture of Zn(NO 3 ) 2 and L 1 -Na 4 with 1,2-dioleoyl-sn-glycero-3-phosphate sodium salt (DOPA) in the Triton X-100/1-hexanol/cyclohexane/water reverse microemulsion at room temperature for 30 min. Transmission electron microscopy (TEM) images of 1 demonstrated the formation of uniform spherical nanoparticles with a diameter of 23.1±7.1 nm ( Fig. 1b and Supplementary Figs 4a and 5a ), which matched the hydrodynamic diameter of 21.3±6.3 nm as measured by dynamic light scattering (DLS). Zn(II) bisphosphonate NCP containing the oxaliplatin prodrug, 2 , was similarly prepared by reacting Zn(NO 3 ) 2 , L 2 -Na 4 , and DOPA to afford slightly larger particles with a diameter of 26.9±10.7 nm by TEM ( Fig. 1e and Supplementary Figs 4d and 5c ) and 28.7±9.2 nm by DLS ( Fig. 1g ). Prodrug loadings in 1 and 2 were determined by inductively coupled plasma-mass spectrometry (ICP-MS) to be 48±3 and 45±5 wt%, respectively. DOPA-free 1 and 2 were also synthesized to determine DOPA amounts on the surface of NCP particles ( Supplementary Fig. 6 and Supplementary Table 1 ). 1 and 2 are amorphous by powder X-ray diffraction and have empirical formulae of Zn 3.5 · L 1 ·DOPA 0.3 ·(OH) 2.7 ·3H 2 O and Zn 3.5 · L 2 ·DOPA 0.3 ·(OH) 2.7 ·5H 2 O ( Supplementary Fig. 7 and Supplementary Methods ). The complete removal of Triton X-100 after washing was confirmed by high-performance liquid chromatography ( Supplementary Fig. 8 ). NCPs 1 and 2 were further pegylated to afford 1P and 2P by mixing a tetrahydrofuran solution (0.276 ml) of 1,2-dioleoyl-sn-glycero-3-phosphocholine (DOPC, 0.54 μmol), cholesterol (0.54 μmol) and 1,2-distearoyl-sn-glycero-3-phosphoethanolamine- N -[methoxy(polyethylene glycol)-2000] (DSPE-PEG 2k , 0.27 μmol) in a 4:4:2 molar ratio and NCP nanoparticles (0.5 mg) to 0.5 ml of 30% (v/v) ethanol/H 2 O at 50 °C. This pegylation protocol takes advantage of the hydrophobic/hydrophobic interactions between DOPA and DOPC/cholesterol/DSPE-PEG 2k to form a self-assembled, asymmetric lipid bilayer on the NCP surface. Cholesterol is abundant in the membrane of animal cells at a molar concentration of 20–50%. The ability of cholesterol to order, condense and stabilize a membrane structure has been extensively studied both experimentally and computationally [42] , [43] . Cholesterol (40 mol%) was added to the present formulations to stabilize the lipid bilayers. On evaporating tetrahydrofuran and cooling to room temperature, the particle suspension was used for cell and mouse studies. Although the TEM images did not show differences in size for the NCPs after pegylation, DLS measurements in 11.8 mM phosphate-buffered saline (PBS) indicated that the hydrodynamic diameters of pegylated NCPs are 15–17 nm bigger than the particle diameters determined by TEM ( Fig. 1c,f and Supplementary Figs 4b,e and 5b,d ), which can be attributed to the lipid layer of DOPC/cholesterol/DSPE-PEG 2k on the particle surfaces as well as swelling of the NCP cores in PBS [44] . DLS diameters of 1 P and 2 P are 41.2±9.1 and 44.1±6.1 nm, respectively, and the ζ potentials measure neutral in PBS at pH 7.4 ( Table 1 ). All of the synthetic steps have been scaled up to hundreds of milligram scales with standard laboratory glassware (500 ml), and the particles from hundreds of batches have shown consistent drug loadings, particle shapes and sizes, and other characteristics, including ζ potential, particle stability, lipid coating and pegylation, and pK properties. The small sizes and near-neutral ζ potentials of the pegylated NCPs make them excellent candidates for in vivo applications [11] , [45] , [46] . Pegylated Zn-pyrophosphate particles with a DLS diameter of 51.6±12.2 nm and a ζ potential of −1.2±0.7 mV were similarly synthesized (see Supplementary Fig. 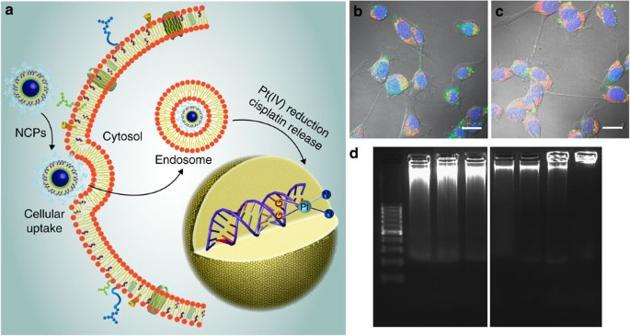Figure 2: Proposed uptake pathways of NCPs and the mechanism of action. (a) Schematic showing endocytosis of NCPs and subsequent reduction ofL1orL2by intracellular reducing agents, such as glutathione, to release cytotoxic cisplatin and oxaliplatin. (b) Confocal fluorescence images of CT26 cells incubated with1P’(b) and2P’(c), showing particle internalization (red channel) and cell apoptosis (green channel). Scale bars, 20 μm. The orange colour is due to the overlap of red and green colour. (d) Gel electrophoresis images showing DNA damage induced by NCPs. From left to right: DNA marker,1P, cisplatin, cisplatin prodrug,2P, oxaliplatin, oxaliplatin prodrug and Zn Control. 9 , Supplementary Table 2 and Supplementary Methods ) and used as a control to test the safety of NCP particle excipients in animal studies. Table 1 Physicochemical properties of NCPs. Full size table Cytotoxicity of NCPs via endocytosis and triggered release L 1 and L 2 ligands are stable under typical physiological conditions, such as those circulating in the blood, but are expected to be readily reduced in more reducing environments, such as within tumour tissues and inside cancer cells. 195 Pt NMR studies indicated that L 1 and L 2 can be instantaneously reduced by 5 mM cysteine to afford cisplatin and oxaliplatin analogue ( Supplementary Fig. 10 and Supplementary Methods ). The in vitro stability of 1P and 2P was evaluated in both PBS buffer with bovine serum albumin and PBS buffer supplemented with 10% fetal bovine serum at 37 °C. Particle sizes remained unchanged over 20 h, thus showing the excellent colloidal and chemical stability of these particles ( Supplementary Fig. 11 and Supplementary Methods ). We also investigated the release kinetics of NCPs in cell culture medium supplemented with 10% fetal bovine serum at 37 °C. The release kinetics is drastically different among lipid-coated, pegylated NCPs and bare particles ( Supplementary Fig. 12 ). The release rate for 1P and 2P was significantly slowed down after pegylation and no burst release was observed, thus demonstrating the effectiveness of the coating strategy. Less than 10% of drug was released from 1P and 2P after incubation at 37 °C for 72 h, as compared with over 50% of drug release for the bare particles during the first 2 h. The Zn release is faster than the drug release from 1P and 2P , probably due to the smaller sizes of Zn ions and thus more facile diffusion through the lipid membrane. The addition of 5 mM cysteine sped up the release of bare NCPs significantly, suggesting the ability to trigger the release of drugs via reductive degradation of NCPs. In contrast, cysteine did not enhance the drug release from 1P and 2P , presumably due to its inability to cross the lipid bilayer. We hypothesized that NCPs can enter cancer cells via endocytosis and readily release cisplatin or oxaliplatin analogue via reduction of L 1 and L 2 by intracellular reducing agents such as glutathione ( Fig. 2a ). 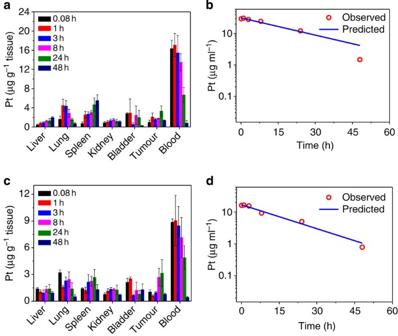Figure 3: Pharmocokinetic and tissue distribution studies of NCPs. Tissue distributions of1P(a) and2P(c) z at time points of 5 min, 1, 3, 8, 24 and 48 h after i.v. injection of corresponding nanoparticles. Data are expressed as means±s.d. (n=3). Observed and fitted time-dependent Pt concentrations in plasma following1P(b) and2P(d) administration. To track the cell internalization of NCPs, we doped 1P and 2P with rhodamine B, an excellent optical imaging agent, by simply adding a small fraction of rhodamine B during the NCP synthesis to afford rhodamine B-doped 1P (denoted as 1P ′) and 2P (denoted as 2P′ ) ( Supplementary Figs 13–15 , Supplementary Table 3 and Supplementary Methods ). Confocal laser scanning microscopy (CLSM) results showed that 1P′ and 2P′ (red fluorescence) were efficiently internalized into the cytoplasm of CT26 cells to induce cell apoptosis as evidenced by the TdT-mediated dUTP nick end-labelling (TUNEL) assays (green fluorescence) ( Fig. 2b,c , Supplementary Fig. 16 and Supplementary Methods ). Furthermore, the presence of the characteristic DNA ladder in cells incubated with 1P , cisplatin, cisplatin prodrug ( L 1 ), 2P , oxaliplatin and oxaliplatin prodrug ( L 2 ), rather than cells incubated with Zn Control indicated that NCPs induced severe DNA damage and cell apoptosis with an efficiency similar to free drugs ( Fig. 2d and Supplementary Methods ). In line with the DNA ladder experiment results, cell viability assays against CT26, H460 and AsPC-1 cancer cell lines gave similar IC 50 values (inhibit cell growth by 50%) for NCPs when compared with their corresponding free drugs ( Supplementary Fig. 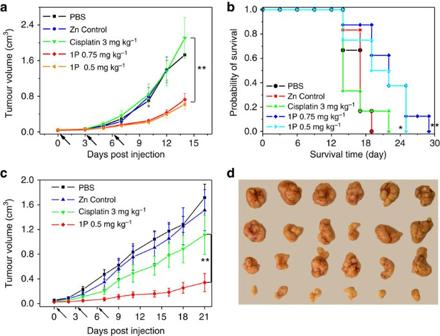Figure 4:In vivoantitumour activity evaluation of 1P. (a)In vivotumour growth inhibition curves for PBS, Zn Control, free cisplatin and1Pon the s.c. C26 tumour model. Cisplatin (dose, 3 mg kg−1) and1P(dose, 0.75 or 0.5 mg kg−1) were administered on day 0, 3, 6. (b) Kaplan–Meier plots showing the percentage of animals remaining in the study with the s.c. C26 tumour model. (c)In vivotumour growth inhibition curves for PBS, Zn Control, free cisplatin and1Pon the s.c. H460 tumour model. Cisplatin (dose, 3 mg kg−1) and1P(dose, 0.5 mg kg−1) were administered on day 0, 3 and 6. Data are expressed as means±s.e.m. (n=6–8), *P<0.05, **P<0.01, ***P<0.001. (d) Photos of resected H460 tumours from various groups. From top to bottom: PBS, Zn Control, free cisplatin and1P. 17 , Supplementary Table 4 and Supplementary Methods ). Finally, we investigated the mechanisms involved in the internalization process by using several uptake inhibitors, including chlorpromazine, genistein, methyl-β-cyclodextrin, wortmannin and NaN 3 ( Supplementary Fig. 18 and Supplementary Methods ). We also used Lysotracker Green to stain the endosomal/lysosomal compartments and chlorea toxin subunit B to mark caveolae-mediated endocytosis ( Supplementary Fig. 19 and Supplementary Methods ). The results obtained from these experiments suggested that the internalization pathway of NCP particles was energy-dependent, clathrin-mediated, caveolae-mediated and lipid-raft-mediated endocytosis rather than via macropinocytosis. Figure 2: Proposed uptake pathways of NCPs and the mechanism of action. ( a ) Schematic showing endocytosis of NCPs and subsequent reduction of L 1 or L 2 by intracellular reducing agents, such as glutathione, to release cytotoxic cisplatin and oxaliplatin. ( b ) Confocal fluorescence images of CT26 cells incubated with 1P’ ( b ) and 2P’ ( c ), showing particle internalization (red channel) and cell apoptosis (green channel). Scale bars, 20 μm. The orange colour is due to the overlap of red and green colour. ( d ) Gel electrophoresis images showing DNA damage induced by NCPs. From left to right: DNA marker, 1P , cisplatin, cisplatin prodrug, 2P , oxaliplatin, oxaliplatin prodrug and Zn Control. Full size image In vivo pK studies of pegylated NCPs We conducted pK studies on 1P and 2P to determine their blood circulation profiles and biodistributions. The plasma Pt concentration (Cp) versus time data were fitted best by a one-compartment model with nonlinear elimination in both cases ( Fig. 3 ). Circulation half-lives of 1P and 2P were determined to be 16.4±2.9 and 12.0±3.9 h, respectively ( Table 2 ). Area under curves were more than 40-fold greater than the reported values of free cisplatin and oxaliplatin [47] , [48] . 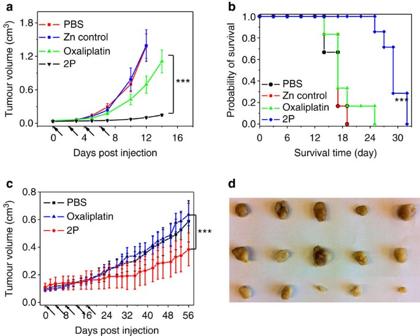Figure 5:In vivoantitumour activity evaluation of 2P. (a)In vivotumour growth inhibition curves for PBS, Zn Control, oxaliplatin and2Pon the s.c. C26 tumour model. Oxaliplatin (dose, 5 mg kg−1) and2P(dose, 2 mg kg−1) were administered on day 0, 2, 4 and 6. (b) Kaplan–Meier plots showing the percentage of animals remaining in the study with the s.c. C26 tumour model. (c)In vivotumour growth inhibition curves for PBS, free oxaliplatin and2Pon the s.c. AsPC-1 tumour model. Oxaliplatin (dose, 5 mg kg−1) and2P(dose, 2 mg kg−1) were administered on day 0, 4, 8, 12 and 16. Data are expressed as means±s.e.m. (n=5–8), *P<0.05, **P<0.01, ***P<0.001. (d) Photos of resected AsPC-1 tumours from various groups. From top to bottom: PBS, oxaliplatin and2P. The long circulation half-lives of 1P and 2P determined by Pt concentrations were consistent with those determined by Zn concentrations in the blood ( Supplementary Figs 20 and 21 , Supplementary Table 5 and Supplementary Discussion 1 ). Thus, 1P and 2P were cleared from the circulation much more slowly than their free drug counterparts. Figure 3: Pharmocokinetic and tissue distribution studies of NCPs. Tissue distributions of 1P ( a ) and 2P ( c ) z at time points of 5 min, 1, 3, 8, 24 and 48 h after i.v. injection of corresponding nanoparticles. Data are expressed as means±s.d. ( n =3). Observed and fitted time-dependent Pt concentrations in plasma following 1P ( b ) and 2P ( d ) administration. Full size image Table 2 Pharmacokinetic parameters for NCPs in CT26 colon tumour-bearing mice. Full size table We also performed pK studies on L 1 -H 4 and L 2 -H 4 as controls for 1P and 2P , respectively ( Supplementary Figs 22 and 23 ). There was significant amount of Pt in the kidney and bladder for L 1 -H 4 and L 2 -H 4 at the 5-min time point, indicating the renal clearance of the prodrugs. A typical biphasic blood circulation profile was observed for both L 1 -H 4 and L 2 -H 4 . The plasma Pt concentration versus time data were fitted best by a two-compartment model in both cases ( Supplementary Figs 22m and 23i ). 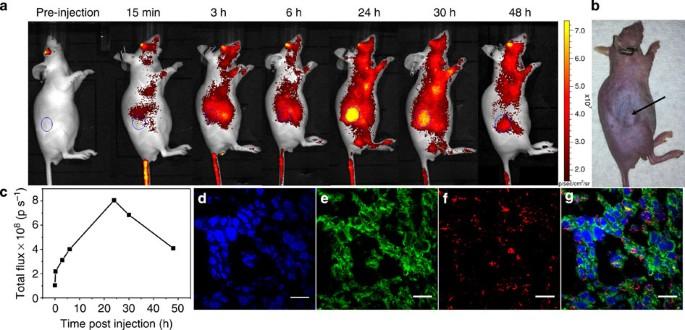Figure 6:In vivofluorescence imaging. (a) Time-dependent fluorescence images of CT26 tumour-bearing mouse showing increasing tumour contrast due to the accumulation of Ce6-1Pinside the tumour. (b) Digital camera image of the same mouse showing the tumour position. (c) Measurements of the fluorescence intensity of the tumour region (circular regions of interest shown in (a)). (d–g) Confocal fluorescence images of CT26 tumour cells. Channels are: DAPI nuclear stain (blue), apoptosis by TUNEL assays (green) and Chlorin e6 from the particles (red). Scale bars, 20 μm. Area under curve values of L 1 -H 4 and L 2 -H 4 were estimated to be 10.8±3.1 and 13.4±2.5 μg ml −1 × h, respectively, which are 70 and 22 times lower than those of 1P (753±42.8 μg ml −1 × h) and 2P (292±32.1 μg ml −1 × h), respectively ( Supplementary Table 6 ). In addition to slow plasma clearance, tissue distribution studies also showed that 1P and 2P were able to avoid uptake by the mononucleosis phagocytosis system (MPS), as judged by the low % ID g −1 (ID stands for injected dose) in the liver, spleen and kidney. This kind of biodistribution was not observed for non-pegylated NCPs. The pK study of non-pegylated 1 showed the deposition of significant amount of injected particles in the liver and spleen (see Supplementary Fig. 22 ). In contrast, the majority of the ID of NCPs 1P and 2P remained in the blood after 24 h, and tumour accumulation of the drug at the 24 h time point approached 8.3±2.8% ID g −1 for 1P and 10.8±5.9% ID g −1 for 2P . In comparison, the highest value of tumour accumulation for non-pegylated 1 was only 1.2±2.8% ID g −1 . To further confirm the stability of NCPs in the blood, we performed ultrafiltration on mice plasma samples obtained at 5 min and 1 h after intravenous (i.v.) injection of 1P and 2P . At the 5-min time point, the ultrafiltrates have 0.88±0.4% ID and 0.43±0.2% ID of Pt for 1P and 2P , respectively, as compared with 83.8±6.6 ID and 63.1±3.4% ID of Pt in the blood circulation for 1P and 2P , respectively. At the 60-min time point, the ultrafiltrates have 2.75±1.6 ID and 2.23±1.0% ID of Pt for 1P and 2P , respectively, as compared with 87.6±9.2 ID and 64.4±21.2% ID of Pt in the blood circulation for 1P and 2P , respectively ( Supplementary Table 7 and Supplementary Methods ). These results indicate that NCPs remain intact in blood circulation, with only a negligible amount of small molecule Pt drugs released in circulation. The NCPs thus possess exceptionally high drug loadings, ideal particle sizes and surface charges, excellent pKs, and trigger release properties to make them excellent vehicles for the selective delivery of cisplatin and oxaliplatin to cancer cells in vivo . In vivo toxicity We examined the maximum tolerated dose (MTD) of 1P and 2P after a single i.v. injection to female Balb/c mice. The MTD was determined based on the group that all mice survived and did not lose over 20% weight. All mice that received Zn Control at five times higher particle dose showed normal weight gain. Dose of 1P at 3 mg kg −1 and dose of 2P at 8 mg kg −1 were well tolerated by the mice, resulting in no death or over 20% weight loss. We conclude that the MTD is ⩾ 3 mg kg −1 for 1P and ⩾ 8 mg kg −1 for 2P ( Supplementary Fig. 24 and Supplementary Methods ). In vivo efficacy studies of pegylated NCPs Three tumour xenograft models, murine colon adenocarcinoma 26 (CT26), H460 human non-small cell lung cancer and AsPC-1 human pancreatic cancer were employed to assess the in vivo antitumour activity of pegylated NCPs. The CT26 colon cancer mouse model has been extensively used to study anticancer efficacy of liposomal and polymeric nanoparticles that carry cisplatin and oxaliplatin [16] , [47] , [49] . We further validated the anticancer activity of 1P using subcutaneous (s.c.) mouse xenografts of the H460 cancer because cisplatin is the first-line treatment for non-small cell lung cancer in the clinic [20] , [50] , [51] , [52] . As oxaliplatin has showed promising results on pancreatic cancer in clinical trials, we used mouse s.c. xenografts of the AsPC-1 pancreatic cancer to ascertain the anticancer activity of 2P [16] , [53] , [54] , [55] . Antitumour activity in CT26 cancer model The antitumour activity of 1P and 2P was first evaluated on a CT26 tumour model. All doses were based on free cisplatin and oxaliplatin equivalents. CT26 tumour-bearing mice were treated by i.v. injection of free cisplatin at the 3 mg kg −1 dose or 1P at doses of 0.75 or 0.5 mg kg −1 every 3 days for three times (q3d × 3). As shown in Fig. 4a , treatment with 0.75 mg kg −1 of 1P resulted in significantly higher antitumour activity (log growth rate of 0.21; P =0.0091) compared with treatment with free cisplatin at the 3 mg kg −1 dose (log growth rate of 0.28). The antitumour efficacy of 0.5 mg kg −1 of 1P was also significantly higher ( P =0.0002) when compared with the free cisplatin group. No differences were observed between the two 1P -treated groups (P>0.1). 1P is thus at least six times more potent than free cisplatin in treating CT26 tumour-bearing mice. Figure 4: In vivo antitumour activity evaluation of 1P. ( a ) In vivo tumour growth inhibition curves for PBS, Zn Control, free cisplatin and 1P on the s.c. C26 tumour model. Cisplatin (dose, 3 mg kg −1 ) and 1P (dose, 0.75 or 0.5 mg kg −1 ) were administered on day 0, 3, 6. ( b ) Kaplan–Meier plots showing the percentage of animals remaining in the study with the s.c. C26 tumour model. ( c ) In vivo tumour growth inhibition curves for PBS, Zn Control, free cisplatin and 1P on the s.c. H460 tumour model. Cisplatin (dose, 3 mg kg −1 ) and 1P (dose, 0.5 mg kg −1 ) were administered on day 0, 3 and 6. Data are expressed as means±s.e.m. ( n =6–8), * P <0.05, ** P <0.01, *** P <0.001. ( d ) Photos of resected H460 tumours from various groups. From top to bottom: PBS, Zn Control, free cisplatin and 1P . Full size image We also determined the efficacy of 2P on CT26 tumour-bearing mice. Mouse xenografts of CT26 tumour were treated i.v. with free oxaliplatin at the 5 mg kg −1 dose or 2P at the 2 mg kg −1 dose four times every other day (q2d × 4). The 2P -treated group gave a log growth rate of 0.13, which was significantly more active ( P =0.0002) than the oxaliplatin-treated group with a log growth rate of 0.26 ( Fig. 5a ). Figure 5: In vivo antitumour activity evaluation of 2P. ( a ) In vivo tumour growth inhibition curves for PBS, Zn Control, oxaliplatin and 2P on the s.c. C26 tumour model. Oxaliplatin (dose, 5 mg kg −1 ) and 2P (dose, 2 mg kg −1 ) were administered on day 0, 2, 4 and 6. ( b ) Kaplan–Meier plots showing the percentage of animals remaining in the study with the s.c. C26 tumour model. ( c ) In vivo tumour growth inhibition curves for PBS, free oxaliplatin and 2P on the s.c. AsPC-1 tumour model. Oxaliplatin (dose, 5 mg kg −1 ) and 2P (dose, 2 mg kg −1 ) were administered on day 0, 4, 8, 12 and 16. Data are expressed as means±s.e.m. ( n =5–8), * P <0.05, ** P <0.01, *** P <0.001. ( d ) Photos of resected AsPC-1 tumours from various groups. From top to bottom: PBS, oxaliplatin and 2P . Full size image The Kaplan–Meier survival plots of treated mice are shown in Figs 4b and 5b , and the results of the Log-rank tests are listed in Supplementary Table 8 , whereas the median survival time (MST) and percentage increased life span (ILS (%)) for each treatment group are summarized in Supplementary Table 9 . 1P- treated mice showed an ILS of 29.4% and 36.8% compared with the control group. 2P showed the largest survival benefit for CT26 tumour-bearing mice with an impressive ILS of 77.9%. In all of the experiments, CT26 tumour-bearing mice were also injected with Zn Control particles at five times higher doses of Zn and lipid components. The Zn control particles did not lead to any tumour suppression, demonstrating the lack of cytotoxicity of the carrier components. Although an average weight loss of 5–10% was observed in NCP-treated groups on day 10th, the mice quickly started to regain the weight once the treatments were finished. No significant difference in weight was observed between NCP and free drug-treated groups at the end of these studies. Antitumour activity in H460 cancer model H460 tumour-bearing mice were treated with i.v. injections of free cisplatin at a 3 mg kg −1 dose or 1P at a 0.5 mg kg −1 dose three times every 3 days (q3d × 3). The 1P- treated group gave a log growth rate of 0.10, which showed significantly greater tumour growth inhibition compared with free cisplatin that had a log growth rate of 0.16 ( P =0.0048, Fig. 4c ). No significant body weight loss was observed in mice over the course of this study ( Supplementary Fig. 25 ). Photos of resected H460 tumours from various groups confirmed that 1P significantly retarded tumour growth ( Fig. 4d ). Antitumour activity in AsPC-1 cancer model Subcutaneous AsPC-1 mouse xenografts were treated with i.v. injections of free oxaliplatin at a 5 mg kg −1 dose or 2P at a 2 mg kg −1 dose five times every 4 days (q4d × 5). The 2P -treated group exhibited significantly higher tumour growth inhibition (with a log growth rate of 0.017) than the free oxaliplatin-treated group (with log growth rate of 0.036, P <0.001). Photos of resected AsPC-1 tumours from various groups confirmed the much enhanced tumour growth inhibition by 2P over free oxaliplatin ( Fig. 5d ). Although ~10% weight loss was observed for mice treated with 2P after the fifth dose on day 18, these mice regained their weight once the treatment was finished. There was no significant difference in weight between 2P- and free oxaliplatin-treated groups at the end of the study ( Supplementary Fig. 25 ). Histopathology analysis and blood chemistry of treated mice Tumour growth inhibition curves and survival benefit analyses clearly indicate that pegylated NCPs are much more effective than their free drugs at treating s.c. xenografts of CT26, H460 and AsPC-1 cancers. Significantly higher tumour growth inhibition and survival benefits were achieved at 16% dose of 1P and 40% dose of 2P in terms of free drug equivalents. A histopathology analysis of the resected tumours confirmed the antitumour potency of NCP particles ( Supplementary Figs 26 and 27 ). Both the untreated and free drug-treated tumours comprised large regions of viable tumour cells, while mice that received NCP nanoparticle treatment had tumours with much larger necrotic areas. In addition, no noticeable histopathological changes were observed for the liver, kidney, lung and spleen in mice treated with pegylated NCP particles ( Supplementary Figs 28 and 29 ), indicating a lack of general toxicity to normal tissues. The toxicity of the NCPs after 0.75 mg kg −1 of 1P q3d × 3 and 2 mg kg −1 of 2P q2d × 4 doses were quantitatively assessed further by examining mouse blood chemistry at 48 h and 5 days after the last dose of treatment. No substantial changes of blood urea nitrogen, creatinine, aspartate aminotransferase or alanine aminotransferase were observed during the time period and all values were within the normal range ( Supplementary Table 10 ). Immunoglobulin E levels, which are correlated with the hypersensitivity to platinum drugs, were also determined after chemotherapy. No significant difference was observed between mice treated with NCPs and mice treated with saline control ( Supplementary Table 11 and Supplementary Methods ). NCP tumour accumulation and in vivo apoptosis induction Chlorin e6-doped NCPs were similarly synthesized (denoted as Ce6- 1P and Ce6- 2P ) and used for the imaging study ( Supplementary Figs 30 and 31 , Supplementary Table 12 and Supplementary Methods ). We conducted whole-body fluorescence imaging on CT26 tumour-bearing mice with Ce6- 1P to visualize and ascertain its enhanced tumour accumulation. When the tumour size reached around 100 mm 3 , mice were i.v.injected with Ce6- 1P at a dose equivalent to 6 mg kg −1 cisplatin. Whole-body imaging was performed before i.v. injection, 15 min, 3 h, 6 h, 24 h, 30 h and 48 h after injection. A sustained systemic distribution of Ce6- 1P was observed after particle injection, indicating the ability of Ce6- 1P to effectively avoid particle opsonization and removal by the MPS. Furthermore, optical signals of tumours were clearly enhanced at 24 and 48 h post injection ( Fig. 6a ). At the 24-h time point, the fluorescence intensity of the tumour region is eight times higher than that of pre-injection. The impressive passive targeting of tumours by Ce6- 1P can thus be attributed to its prolonged circulation times, which significantly enhance the permeability and retention of the nanoparticles in tumours. Figure 6: In vivo fluorescence imaging. ( a ) Time-dependent fluorescence images of CT26 tumour-bearing mouse showing increasing tumour contrast due to the accumulation of Ce6- 1P inside the tumour. ( b ) Digital camera image of the same mouse showing the tumour position. ( c ) Measurements of the fluorescence intensity of the tumour region (circular regions of interest shown in ( a )). ( d – g ) Confocal fluorescence images of CT26 tumour cells. Channels are: DAPI nuclear stain (blue), apoptosis by TUNEL assays (green) and Chlorin e6 from the particles (red). Scale bars, 20 μm. Full size image We also carried out CLSM imaging of dissected tumour tissues to ascertain the enhanced uptake of pegylated NCPs and induced apoptosis of cancer cells in vivo . Five-micrometre-thick frozen sections of tumours were prepared and fixed with 4% (w/v) paraformaldehyde at 4 °C for 45 min. Tumour sections were stained with DAPI (4′,6-diamidino-2-phenylindole) and marked by TUNEL. Significant fluorescence from chlorin e6 (red) and TUNEL (green) was observed in the confocal images ( Fig. 6 ), indicating the ability of these particles to enter cancer cells and induce apoptosis in vivo . It is noted that the fluorescence signals from NCPs were uniformly distributed throughout the entire tumour section at 24 h post injection, suggesting deep tumour penetration of NCPs. In addition to deeper tumour penetration, the apoptosis signals can be seen in areas without particles, which was explained in a recent report to be a result of the ‘neighbouring effect’, which is unique to rapidly proliferating cancer cells such as CT26 cells [56] . The microdistributions of NCP particles in the lung, spleen, liver and kidney were also assessed at 24 h post injection ( Supplementary Fig. 32 ). Nanoparticles exhibit interesting properties that make them ideally suited for cancer imaging and drug delivery [57] . In particular, when compared with their small molecule counterparts, nanotherapeutics can have prolonged blood circulation times to allow for enhanced drug deposition in tumours by taking advantage of the enhanced permeability and retention (EPR) effect due to leaky vasculatures in tumour tissues [12] . However, most of the current nanoparticle platforms are either pure organic (such as liposomes, polymeric micelles, organic polymers and dendrimers) or inorganic (such as metal, metal oxide and mesoporous silica), and they each have strengths and weaknesses. We became interested in developing NCPs with the aim of combining strengths of both inorganic and organic systems into the same platform [33] , [58] , [59] , [60] , [61] . The advantages of using NCPs for drug delivery can be multi-fold. First, NCP formulations can provide unprecedentedly high drug loadings; hence, minimum amounts of excipients are co-delivered to cancer cells. Second, the compositions, shapes and sizes of the NCPs can be tuned by altering synthetic conditions to maximize their delivery efficiency. Third, NCPs are intrinsically biodegradable as a result of relatively labile metal-ligand bonds. Finally, the surface of NCPs can be further modified to impart biocompatibility and targeting efficacy. As the surface properties of NCPs mostly dictate how they interact with cell milieus, proper surface chemistry needs to be employed to make NCPs a suitable drug delivery platform for cancer therapy in vivo . In this work, we used the well-established lipid-coating strategy to stabilize NCPs and to prolong their blood circulation times. Liposomes were first proposed as a drug delivery vehicle for cancer chemotherapy in 1974 (ref. 62 ) and this concept became a reality when the liposomes were further functionalized with a corona of polyethyleneglycol (PEG) [63] . The hydrated PEG coating endows long circulating property to the liposomes by inhibiting protein adsorption and opsonization, leading to enhanced drug deposition in tumours via the EPR effect [64] . The NCP particles were synthesized in the presence of DOPA, and on washing with ethanol and tetrahydrofuran (THF), afforded monodisperse particles with a monolayer of DOPA coating via Zn–phosphate interactions between NCPs and DOPA molecules and hydrophobic–hydrophobic interactions among DOPA molecules. The NCPs were further coated with DOPC, cholesterol and DSPE-PEG 2k in a 4:4:2 molar ratio to lead to self-assembled, asymmetric lipid bilayers via hydrophobic/hydrophobic interactions between DOPA and DOPC/cholesterol/DSPE-PEG 2k . Importantly, the NCP core allows the use of a very high molar ratio (20 mol%) of DSPE-PEG 2k without destabilizing the lipid bilayer. In comparison, liposomes become unstable when the PEG molar ratios exceed 5 mol%, and most of the currently developed or clinically used liposomes have ~5 mol% of PEG in lipid composition, including DOXIL [65] , SPI-77 (ref. 47 ) and Porphysome [66] . As a result of the PEG coating at such a high molar ratio, NCPs 1P and 2P exhibit prolonged blood circulation times and enhanced deposition of the platin drugs in tumour tissues. When compared with liposomal formulations such as SPI-77 and Lipoplatin, NCPs have much higher drug-to-lipid weight ratios of over 1:1. The drug-to-lipid weight ratio is 1: 70 for SPI-77 and 1:10 for Lipoplatin [67] . Despite its superior pK properties, SPI-77 did not demonstrate enhanced therapeutic efficacy over cisplatin in several tumour models due to the lack of cisplatin release in tumour tissue [68] , [69] . As an example of polymer drug conjugates, ProLindac had a very high MTD of >250 mg kg −1 in mice, but also suffered from poor drug release due to covalent attachment of the oxaliplatin prodrug to the polymer backbone [48] , [70] . NCPs have similar particle sizes and drug loadings to polymeric micelle systems, such as CCDP/m and DACHPt/m, but are able to achieve comparable or better tumour inhibition by using much lower doses (0.5 mg kg −1 of cisplatin and 2 mg kg −1 of oxaliplatin for NCPs versus 4 or 5 mg kg −1 of cisplatin and 8 mg kg −1 of oxaliplatin for polymeric micelle systems). This difference in performance can be attributed to the unique drug retention and release properties of NCPs. We hypothesize that on endocytosis, 1P and 2P can lose some of the lipid coatings to expose bare NCP particles, which will degrade to release cisplatin and oxaliplatin under reducing environments. Detailed comparisons of NCPs with selected formulations are summarized in Supplementary Table 13 . The three tumour models we examined in this work responded quite differently to cisplatin and oxaliplatin treatment. Colon cancer is more sensitive to oxaliplatin treatment than cisplatin treatment; thus, the observed log growth rate of 0.13 after the treatment of 2P is significantly slower than the growth rate of 0.21 obtained after the treatment of 1P . Among the three models, CT26 is the most aggressive while AsPC-1 is the least aggressive. However, as pancreatic cancer is of the least permeable tumour, many attempts made to date to treat pancreatic cancer have failed. Only those particles with a small size to penetrate deeply into pancreatic tumour can elicit an antitumour effect. The in vivo results show that NCPs with a particle size of <50 nm are not only effective on highly permeable tumours such as CT26 and H460, but also exert a high tumour growth inhibition effect on pancreatic tumour. This observation is consistent with the recent findings by Kataoka and coworkers [16] . In summary, we have developed novel NCP-based nanotherapeutics that show significant and numerous advantages over existing systems. First, the self-assembly of NCPs is carried out under mild conditions without using specialized equipment, making the NCP synthesis highly scalable. Second, particle size and drug loading were found to be very consistent from batch to batch among the several hundreds of batches of NCP particles synthesized. Third, the NCP platform carries very high drug loadings, which not only minimizes the amount of excipients that are co-delivered but also alleviates the potential aggregation issue often encountered by particles with modest drug loadings. Fourth, a particle size of 30–50 nm and near-neutral surface charge are two of the most desirable characteristics for nanotherapeutics. Small particles have enhanced penetration within tumours [16] , whereas particles with near-neutral surface charge ranging (from −10 to +10 mV) can minimize nonspecific interactions with proteins, self-aggregation and phagocytosis [14] . NCPs effectively avoid MPS uptakes to lead to long circulation times, which is a key prerequisite for passive targeting by the EPR effect. Fifth, we have shown that the excipients used in the NCPs are non-toxic and biocompatible. Sixth, the pegylated NCPs showed no burst release at the initial stage, thus preventing premature drug release before the particles reach tumour sites. Finally, the NCP has a built-in trigger release mechanism to further enhance drug deposition in tumours. With the above attributes, we have successfully demonstrated selective and substantial accumulation of chemotherapeutics with pegylated NCPs in solid tumours via the passive targeting pathways. In in vivo antitumour activity studies using CT26, H460 and AsPC-1 models, we showed that NCPs were significantly more effective than small molecule drugs even with 16.7%–40% of the dose of free drugs. This level of enhanced potency is still rare in the nanomedicine literature, suggesting that NCPs represent a significant breakthrough as a novel and effective drug delivery system for potential translation to the clinic. Materials All of the starting materials were purchased from Aldrich and Fisher, unless otherwise noted, and used without further purification. DOPC, DOPA and DSPE-PEG 2k were purchased from Avanti. Fetal bovine serum was purchased from Hyclone, Logan, UT. RPMI-1640 growth medium, penicillin–streptomycin and PBS were bought from Gibco, Grand Island, NY. 1 H NMR spectra were recorded on a Bruker NMR 400 DRX Spectrometer at 400 MHz and referenced to the proton resonance resulting from incomplete deuteration of deuterated chloroform or dimethyl sulphoxide. 195 Pt NMR spectra were referenced externally using standards of K 2 PtCl 4 in D 2 O ( δ =−1,628 p.p.m.). Ultraviolet–visible absorption spectra were obtained using a Shimadzu UV-2401PC UV–vis Spectrophotometer. Thermogravimetric analyses were performed using a Shimadzu TGA-50 equipped with a platinum pan. A Hitachi 4700 field emission scanning electron microscope (SEM) and a JEM 100CX-II TEM were used to determine particle size and morphology. SEM images of the nanoparticles were taken on glass substrate. A Cressington 108 Auto Sputter Coater equipped with a Au/Pd (80/20) target and MTM-10 thickness monitor was used to coat the sample with ~5 nm of conductive layer before taking SEM images. Size and zeta potential data were collected with a Malvern Zetasizer Nano Zs. A Varian 820-MS ICP-MS was used to determine Mn and Pt concentration. Samples were introduced via a concentric glass nebulizer with a free aspiration rate of 0.4 ml min −1 , a Peltier-cooled double-pass glass spraychamber and a quartz torch. A peristaltic pump carried samples from an SPS3 autosampler (Varian) to the nebulizer. All standards and samples were in 2% HNO 3 , prepared with MilliQ water. HPLC analysis of Triton X-100 was carried out on LC-10AT VP (Shimadzu, Japan) equipped with SPD-M10A VP diode array detector, SIL-10AF auto injector and SCL-10A VP system controller. Column: Dynamax-300A C18 (250 × 4.14 mm, 5 μm) (Rainin Instrument Co. InC., Woburn, MA). Tumour model Female, Foxn1 nu/nu mice were inoculated s.c. with CT26 cells (one million cells per mouse) or H460 cells (five million cells per mouse) or AsPC-1 cells (five million cells per mouse). Antitumour activity studies were performed when tumours were 30–50 mm 3 for CT26 and H460, respectively, and ~100 mm 3 for AsPC-1. Biodistribution studies were performed when the tumours were 100–200 mm 3 . All animal experiments were performed in accordance with the protocol approved by the institutional animal care and use committee at the University of North Carolina and the University of Chicago. Procedures for nanoparticle synthesis A w =7.4 microemulsion was prepared by the addition of 0.2 ml of a 25 mg ml −1 L 1 -Na 4 aqueous solution (obtained by deprotonation with 3 M NaOH) and 0.2 ml of a 100 mg ml −1 Zn(NO 3 ) 2 aqueous solution to separate 5 ml aliquots of a 0.3 M Triton X-100/1.5 M 1-hexanol in cyclohexane mixture while vigorously stirring at room temperature. Twenty microlitres of DOPA solution (200 mg ml −1 in CHCl 3 ) was added to the complex solution and the stirring was continued for 15 min until a clear solution formed. The two microemulsions were combined and the resultant 10 ml microemulsion with w =7.4 was stirred for 30 min. After the addition of 20 ml ethanol, 1 was obtained by centrifugation at 12,000 r.p.m. The resulting pellet was washed once with ethanol and twice with 50% ethanol/THF, and redispersed in THF. Particles were purified by filtration through 200 nm syringe filter. 2 was similarly prepared. General procedures for pegylation Pegylated particles were obtained by adding a THF solution of DOPC, cholesterol (1:1molar ratio), DSPE-PEG 2k (20 mol%) and nanoparticles to 500 μl 30% (v/v) ethanol/H 2 O at 50 °C. THF was completely evaporated and the solution was allowed to cool to room temperature before use. pKs and tissue distributions Mice were injected in the right flank with one million CT26 cells and tumours were allowed to grow until 100 to 200 mm 3 before they received a 3-mg cisplatin or oxaliplatin per kg dose of NCP particles by tail vein injection. Animals were killed (three per time point) at 5 min, 1 h, 3 h, 8 h, 24 h and 48 h after dosing. The liver, lung, spleen, kidney and bladder were excised and kept in dry ice before analysis. Blood was collected by cardiac puncture and kept in heparinized tubes. Organs and blood were digested in concentrated nitric acid for at least 24 h and analysed by ICP-MS. In vivo antitumour activity CT26 cells (one million cells per mouse), H460 cells (five million cells per mouse) or AsPC-1 (five million cells per mouse) were injected s.c. into the right flank of mice. Tumour volume and body weights were measured for individual animals three times weekly in all experiments. Tumour volume was determined by measuring the tumour in two dimensions with calipers and calculated using the formula tumour volume=(length × width 2 )/2. Mice were killed when tumour volume reached the maximum allowed size. MST (day) was defined as the time at which half of the mice had died. The percentage ILS (%) was calculated using the following equation: ILS (%)=[(MST of treated group/MST of control group)−1] × 100. Tissue histopathology evaluation The liver, kidney and tumours were received in a formalin solution. For histology, organs and tumours were placed in labelled cassettes and flushed with water for 20 min. Samples were then transported to the Lineberger Comprehensive Cancer Center Animal Histopathology Core Lab in a 70% ethanol solution where they were pariffinized, cut and haematoxylin and eosin stained. The stained samples were imaged at the UNC Microscopy Services Laboratory using an Olympus BX61 Upright Fluorescence Microscope equipped with Improvision’s Volocity software. Images were captured using a QImaging RETIGA 4000R colour camera. Blood chemistry analysis To test hepatic and renal functions of treated mice, blood was drawn 48 h and 5 days after the last dose of treatment for blood chemistry analyses. Blood samples were centrifuged down at 6,000 r.p.m. for 15 min and the supernatant blood serums were collected and transported to UNC Animal Clinical Laboratory Core Facility for analysis of creatine, blood urea nitrogen, alanine aminotransferase and aspartate aminotransferase levels using Vitros 350 Chemistry System (Ortho Clinical Diagnostics Company, Rochester, NY). In vivo fluorescence imaging CT26 cells were injected s.c. into the right flank of female nude mice. When the tumour size reached around 100 mm 3 , mice were i.v.injected with 1P ’. Whole-body imaging was performed under the IVIS Kinetic Imaging System (Caliper Life Sciences, Hopkiton, MA) with excitation filter of 640 nm and emission filter of 700 nm before i.v. injection, 15 min, 3 h, 6 h, 24 h, 30 h and 48 h after injection. All imaging parameters were kept constant for the whole imaging study. Binning factor=4, exposure time=3 s, f number=2 and field of view=12.5. Region of interest values were recorded using Living Image software as total photon counts per centimetre-squared per steradian (p s −1 cm −2 sr −1 ). Confocal microscopy Tumour was harvested, rinsed in saline and cryofixed in optimal cutting temperature medium. Frozen sections of 5-μm thickness were prepared and fixed with 4% (w/v) paraformaldehyde at 4 °C for 45 min. To visualize cell apoptosis, TUNEL reaction was performed on tumour sections using DNA fragmentation detection kit (Life Technology, USA) according to the manufacturer’s instructions. The nuclei were stained with 10 μg ml −1 of DAPI. Images were captured with an Olympus Fluoview 1,000 CLSM at the University of Chicago Integrated Light Microscopy Facility. Statistical analysis The SAS statistical package (SAS Institute, Inc., Cary, NC) was used for longitudinal data and repeated measurement analysis. SAS procedure PROC MIXED with unspecified covariance structure was used to evaluate treatment and time effects on tumour growth. We fitted mixed models to the tumour growth curve data by a log transformation of tumour volume at each time point and estimated the exponential growth rates. Survival studies were analysed using the Kaplan–Meier and Log-rank tests with Origin. How to cite this article: Liu, D. et al . Self-assembled nanoscale coordination polymers with trigger release properties for effective anticancer therapy. Nat. Commun. 5:4182 doi: 10.1038/ncomms5182 (2014).